Integrated analysis of germline and somatic variants in ovarian cancer We report the first large-scale exome-wide analysis of the combined germline–somatic landscape in ovarian cancer. Here we analyse germline and somatic alterations in 429 ovarian carcinoma cases and 557 controls. We identify 3,635 high confidence, rare truncation and 22,953 missense variants with predicted functional impact. We find germline truncation variants and large deletions across Fanconi pathway genes in 20% of cases. Enrichment of rare truncations is shown in BRCA1 , BRCA2 and PALB2 . In addition, we observe germline truncation variants in genes not previously associated with ovarian cancer susceptibility ( NF1 , MAP3K4 , CDKN2B and MLL3) . Evidence for loss of heterozygosity was found in 100 and 76% of cases with germline BRCA1 and BRCA2 truncations, respectively. Germline–somatic interaction analysis combined with extensive bioinformatics annotation identifies 222 candidate functional germline truncation and missense variants, including two pathogenic BRCA1 and 1 TP53 deleterious variants. Finally, integrated analyses of germline and somatic variants identify significantly altered pathways, including the Fanconi, MAPK and MLL pathways. Ovarian cancer is diagnosed in ~22,000 women annually in the United States. The average 5-year survival is relatively poor at ~44% (ref. 1 ), which is primarily due to late-stage diagnosis. It is currently estimated that 20–25% of women have an inherited germline mutation that predisposes them to ovarian cancer [2] , [3] . New strategies for the prevention and control of ovarian cancer will rely on a thorough understanding of the contributing genetic factors both at the germline and somatic levels. High-throughput sequencing technologies are rapidly expanding our understanding of ovarian cancer biology by providing comprehensive descriptions of genetic aberrations in tumours [4] . The ability to rapidly sequence individual tumour and normal genomes allows for efficient discovery of candidate cancer-causing events and such work is already transforming risk assessment, diagnosis and treatment. For example, targeted sequencing of 21 tumour suppressor genes in 360 cases of ovarian, peritoneal, fallopian tube and synchronous ovarian/endometrial carcinomas recently revealed that 24% of cases harboured germline loss-of-function mutations in 1 of 12 genes: BRCA1 , BRCA2 , BARD1 , BRIP1 , CHEK2 , MRE11A , MSH6 , NBN , PALB2 , RAD50 , RAD51C and TP53 (ref. 3 ). In a different study, the Cancer Genome Atlas (TCGA) consortium analysed somatic alterations in 316 serous ovarian carcinomas, identifying recurrent somatic TP53 mutations in nearly all cases (96%) and finding recurrent somatic mutations in NF1 , BRCA1 , BRCA2 , RB1 and CDK12 in a minority of cases [4] . Such work is deepening our understanding of genes involved in ovarian cancer. Cancer genomics studies have most often focused on independent analyses of either somatic or germline mutations. However, studies that perform sequencing of matched tumour and normal samples have the advantage that data from the somatic and germline genomes can be ascertained and integrated to build a fuller picture of each genome’s contribution to disease. In addition, the rapidly growing number of publicly available exome data sets from non-cancer populations now facilitates rare germline susceptibility variant discovery. Here we describe the somatic and germline mutation spectrum in the tumour and normal exome data from 429 TCGA serous ovarian cancer patients. To identify candidate pathogenic variants, we compare the frequency of germline mutations with those from a large control data set of sequences of post-menopausal women from the Women’s Health Initiative Exome Sequencing Project (WHISP). We identify several novel candidate germline predisposition variants in known ovarian genes (for example, BRCA1 , BRCA2, ATM, MSH3 and PALB2 ) as well as several genes not previously associated with ovarian cancer (for example, ASXL1 , RB1 , NF1 , CDKN2A and EXO1 ). We also characterize patterns of loss of heterozygosity (LOH) in tumour suppressor genes, including BRCA1 , BRCA2 , BRIP1 , ATM , CHEK2 and PALB2 , and identify significantly mutated pathways, including Fanconi anaemia, mitogen-activated protein kinase (MAPK) and mixed lineage leukemia (MLL). These results provide a foundation for future functional and clinical assessment of susceptibility variants in ovarian cancer. Clinical characteristics of samples Of the 429 TCGA cases in this analysis, 90.2% were Caucasian ( n =387), 4.9% were African American ( n =21), 3.5% were Asian ( n =15) and 0.5% ( n =2) were American Indian/Alaska Native. 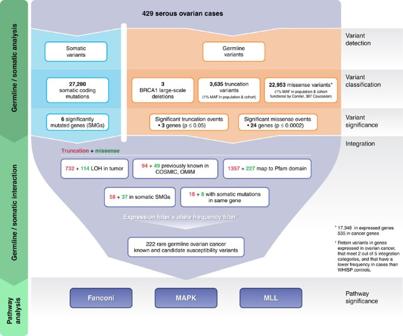Figure 1: Overview of the integrated analysis of germline and somatic variants in 429 TCGA serous ovarian cases. A total of 27,280 somatic mutations were identified, including 6 SMGs (blue shaded area). Germline variants included a total of three BRCA1 large-scale deletions, following filtering of variants with >1% MAF in the population, TCGA ovarian cancer cases and WHISP controls; a total of 3,635 truncation variants and 22,953 missense variants (17,348 in expressed genes) remained for TCGA cases. For WHISP controls, a total of 10,443 truncation and 30,335 missense variants (in expressed genes) remained. After applying the burden test using WHISP exome sequence data, a total of 3 and 24 genes were significantly enriched for truncation events and missense variants, respectively (orange shaded area). The germline–somatic interaction analysis (purple shaded area) that retained variants in expressed genes in ovarian cancer that met two out of five criteria identified a total of 222 candidate germline susceptibility variants. The pathway analysis identified three significant pathways involved in ovarian cancer pathogenesis, Fanconi, MAPK and MLL. Patients were diagnosed between 26 and 89 years (mean 59.4±11.8 years), frequently at late stage (93% at stages 3–4) and 50.8% were deceased at the time of TCGA sample procurement ( Table 1 ). Nineteen of 23 cases with unknown ethnicity information were assigned Caucasian ( n =17) and African ancestry ( n =2) using principal components analysis ( Supplementary Fig. 1 ). We performed systematic germline variant and somatic mutation analyses for the sample set, as illustrated in Fig. 1 . Table 1 Clinical characteristics of TCGA cases. Full size table Figure 1: Overview of the integrated analysis of germline and somatic variants in 429 TCGA serous ovarian cases. A total of 27,280 somatic mutations were identified, including 6 SMGs (blue shaded area). Germline variants included a total of three BRCA1 large-scale deletions, following filtering of variants with >1% MAF in the population, TCGA ovarian cancer cases and WHISP controls; a total of 3,635 truncation variants and 22,953 missense variants (17,348 in expressed genes) remained for TCGA cases. For WHISP controls, a total of 10,443 truncation and 30,335 missense variants (in expressed genes) remained. After applying the burden test using WHISP exome sequence data, a total of 3 and 24 genes were significantly enriched for truncation events and missense variants, respectively (orange shaded area). The germline–somatic interaction analysis (purple shaded area) that retained variants in expressed genes in ovarian cancer that met two out of five criteria identified a total of 222 candidate germline susceptibility variants. The pathway analysis identified three significant pathways involved in ovarian cancer pathogenesis, Fanconi, MAPK and MLL. Full size image Data for 614 samples from the National Heart, Lung, and Blood Institute (NHBLI) Women's Health Initiative Exome Sequencing Project WHISP were used for comparison of genetic variants with TCGA ovarian cancer cases. After extensive quality checks (Methods), 557 Caucasians with an average age of 63.3±7.8 years (range 50–79 years) were selected as controls for downstream ovarian susceptibility variant analysis ( Supplementary Data 1 ). Somatic mutations and significantly mutated genes We analysed somatic mutations in 429 ovarian cancer cases. Of these, 142 were new TCGA cases and 287 cases were previously reported [4] ; the remaining 29 cases reported in that study [4] did not meet our coverage requirement (≥20 × coverage for at least 50% of target exons) and were excluded from this analysis. The average exome-wide coverage for the entire sample set was 68.1 × with 99.5 × and 96.5 × average coverages for BRCA1 and BRAC2 , respectively. We identified 11,479 somatic mutations in the 142 new TCGA cases. All of these mutations were manually reviewed, resulting in a total of 27,280 mutations in 429 cases ( Fig. 1 and Supplementary Data 2 and 3 ). After removing genes with low or no RNA expression evidence from RNA-seq data, the significantly mutated genes (SMGs) identified by MuSiC [5] include those previously reported: TP53 , NF1 , RB1 , CDK12 ( CRKRS) and BRCA1 (ref. 4 ), as well as the new SMG, KRAS ( Supplementary Table 1 ). BRCA2 and RB1CC1 were near significance. We also identified 4 NRAS mutations, 3 NF2 mutations and 3, 8, and 10 mutations in the known tumour suppressor genes: ATR , ATM and APC , respectively. Somatic truncation mutations were also observed in histone modifier genes including the following: ARID1A , ARID1B , ARID2 , SETD2 , SETD4 , SETD6 , JARID1C , MLL , MLL2 and MLL3 as well as the DNA excision repair gene ERCC6 ( Supplementary Data 3 ). Germline variant landscapes and significant germline events We identified germline truncation variants (nonsense, non-stop, splice site and frameshift indels) in 429 matched tumour-normal cases using multiple algorithms [6] , [7] , [8] . After removal of common variants, reference sequence errors and recurrent artifacts, a total of 3,635 high confidence, rare (<1% population minor allele frequency (MAF)) germline truncation variants were identified in 2,214 genes, 115 of which are in 40 known cancer genes ( Fig. 1 , Supplementary Fig. 2 ; Supplementary Data 4 and Methods) [9] . These 115 variants were validated using genomic DNA or a source of whole-genome-amplified DNA that differed from that used for discovery ( Supplementary Data 5 ). We used several approaches to identify known and potentially pathogenic germline missense variants in the Caucasian subset ( Table 1 , n =387). Specifically, a total of 22,953 missense variants in 3,637 genes were predicted to be functionally deleterious by Condel [10] and also had population MAFs <1% in Caucasian data from the 1,000 Genomes, and the current cohorts (TCGA ovarian cancer cases and WHISP exome controls; Fig. 1 , Supplementary Data 6 and Supplementary Fig. 3 ). After limiting our analyses to genes with an average expression Reads Per Kilobase per Million mapped reads (RPKM)>0.5 (Methods), we identified 17,348 missense variants in a total of 2,810 genes in this subset. We processed 557 WHISP samples using the same software tools and filtering strategies and identified 7,889 rare (<1% MAF in the population and cohort) truncation variants and 30,335 rare missense variants defined as functionally deleterious by Condel and in expressed genes ( Supplementary Data 7 and 8 ). Finally, although we performed a genome-wide germline copy-number analysis using single nucleotide polymorphism (SNP) array data, our manual review of the results indicated many false positives with very few passing our review criteria. Therefore, we focused our analysis of copy-number alterations on BRCA1 , BRCA2 and TP53 , coupled with extensive manual review. Here three high-confidence germline deletion events in BRCA1 were identified in three cases (TCGA-36-2539, TCGA-31-1959 and TCGA-23-1028; Fig. 2 ). Two cases (TCGA-31-1959 and TCGA-23-1028) developed ovarian cancer at younger ages (50 and 43 years, respectively); information regarding age of diagnosis for TCGA-36-2539 was not available. 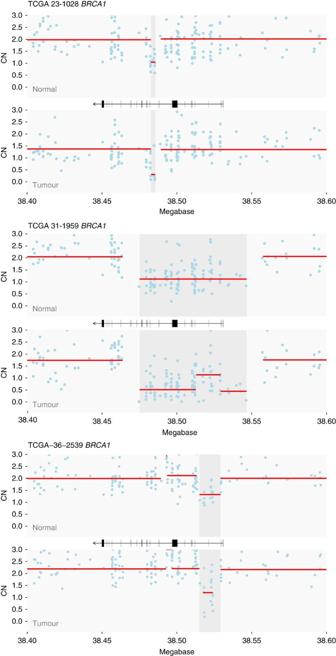Figure 2:Germline copy-number variants inBRCA1. Shown are three germline copy-number deletion variants affectingBRCA1in three ovarian normal tumour pairs. Normal samples appear above the corresponding tumour samples. Red lines indicate normalized copy-number segments based on a minimum of eight probes, and blue dots indicate individual probe intensities from Affymetrix 6.0 SNP arrays within the region. Figure 2: Germline copy-number variants in BRCA1. Shown are three germline copy-number deletion variants affecting BRCA1 in three ovarian normal tumour pairs. Normal samples appear above the corresponding tumour samples. Red lines indicate normalized copy-number segments based on a minimum of eight probes, and blue dots indicate individual probe intensities from Affymetrix 6.0 SNP arrays within the region. Full size image We used a right-tailed cohort allelic sums test (CAST) [11] burden test, CAST greater (personal communication, Q.Z. ), to evaluate expressed genes (Methods) having significant enrichment of rare, potentially pathogenic missense variants in the TCGA Caucasian exomes versus the WHISP control group and the test identified 24 genes that had significant enrichment ( P <0.0002, CAST greater ). As expected, BRCA1 was one of the most significant genes on the list ( P =1.40 E−06, CAST greater ). A total of nine unique BRCA1 rare missense variants were detected in this ovarian cancer cohort; this list included two known pathogenic missense variants (R1699W and G1788V) and three singletons (V772A, L668F and P1637L). It also included one known ovarian cancer susceptibility gene ( FANCM; P =4.04E−06, CAST greater ) as well as three cancer genes ( ARID1A , EGFR and DNMT1 ), not previously implicated in ovarian cancer ( Supplementary Data 6 and 9 ). ARID1A , frequently mutated in endometrial cancer [12] , and EGFR , a prominent oncogene involved in lung cancer [13] and glioblastoma [14] , harboured 10 and 5 rare (≤1% MAF) unique missense variants in this ovarian cancer sample set, respectively. Several other known cancer genes (for example, CREBBP , ASXL1 , EZH2 and BRIP1) were also found to be in the top 100 and with P CAST greater <0.0015. The significance of other top genes such as EEF2K requires additional investigation using larger sample sets. We next focused on comparison of rare germline truncations in cancer genes between TCGA ovarian cases and the WHISP control set. Three known ovarian cancer susceptibility genes were significant at the right-tailed CAST test with P ≤0.05 as the threshold ( BRCA1 ( P =2E−08), BRCA2 ( P =8.89E−06) and PALB2 ( P =0.042)) and two other known ovarian cancer susceptibility genes were among the highest ranked genes, although they did not reach significance ( CHEK2 ( P =0.11) and BRIP1 ( P =0.11)) ( Supplementary Table 2 ). A total of 66 cases had truncations in one of these genes ( Supplementary Data 4 and 5 ). It is noteworthy that we have identified truncation mutations in USP6 , ROPN1L and RYR1 , although their involvements in cancer are unclear. In addition, three truncation variants (T1222fs, Q645* and L258fs) were detected in BLM , a gene recently linked to familial breast cancer [15] . Q645* and L258fs were previously reported in BLMbase ( http://www.bioinf.uta.fi/BLMbase/ ). The distribution of germline and somatic mutations in these genes is shown in Fig. 3 . It is interesting to note that 11 cases had germline truncation variants in multiple cancer genes, including two cases with BRCA1 and BRCA2 variants (diagnosis ages 49 and 55 years), one case with BRCA2 and ERCC3 variants, one with PALB2 and ATM variants and one with BLM and FANCD2 truncation variants. Finally, five cases had germline truncation variants in other genes on the cancer gene list, including: ERCC2 ( n =1), TET2 ( n =1), FANCD2 ( n =2) and NF1 ( n =1) while one case had a germline mutation in RAD51B , which has recently been linked to breast cancer susceptibility [16] and whose family members ( RAD50 , RAD51C and RAD51D ) have previously been implicated in ovarian cancer susceptibility [17] . 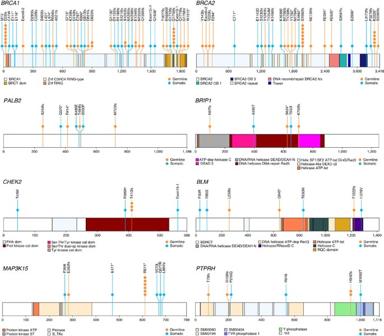Figure 3: Lolliplots showing the distribution of germline truncation variants and somatic mutations. Somatic mutations inBRCA1,BRCA2,PALB2,CHEK2,BRIP1,BLM, MAP3K15andPTPRHare shown in blue and germline truncation variants are in orange. Two known pathogenicBRCA1germline missense variants are also shown (G1788V and R1699W). Figure 3: Lolliplots showing the distribution of germline truncation variants and somatic mutations. Somatic mutations in BRCA1 , BRCA2 , PALB2 , CHEK2 , BRIP1 , BLM, MAP3K15 and PTPRH are shown in blue and germline truncation variants are in orange. Two known pathogenic BRCA1 germline missense variants are also shown (G1788V and R1699W). Full size image When we combined missense and truncation variants in cancer genes for burden testing, known cancer susceptibility genes were among the most significant genes on the list ( BRIP1 (refs 3 , 18 ) and BRCA1 ). In addition, other established/suspected ovarian/breast cancer susceptibility genes were significant, including BRCA2 (ref. 2 ) and NF1 (ref. 19 ); novel genes such as ASXL1 , frequently mutated in myelodysplastic syndromes [20] , myeloproliferative neoplasms [21] and AML [22] ; SETD2 , involved in clear cell renal cell carcinoma [23] ; and MAP3K1 , a newly discovered breast cancer gene [24] , [25] ( Supplementary Data 10 ). Germline variants that have been detected as somatically mutated in cancer might signal functional relevance of these variants. We compared our identified germline truncation and missense variants with those present in the COSMIC and OMIM databases to determine whether any were reported in other studies. Of the 3,635 exome-wide truncation variants, 84 and 10 germline variants matched precisely or within ±5 amino acids to reported variants in COSMIC and OMIM, respectively ( Supplementary Data 11 ). Further analysis of 535 missense variants from cancer genes, using the same criteria applied for truncations, identified 35 and 14 missense events in COSMIC and OMIM, respectively ( Supplementary Data 11 ). For example, the ASXL1 germline variant G1397S that we identified in 6 of 387 ovarian cancer cases versus 2 of 557 WHISP non-cases and the ASXL1 germline variant G643V identified in 1 of 387 cases versus 0 of 557 WHISP non-cases have previously been found to be somatically mutated in haematologic malignancies [26] , [27] . Although there was not an exact match of the germline variant P333L in TET2 in COSMIC (observed in 1 of 387 cases versus 0 of 557 WHISP non-cases), a somatic frameshift mutation, P333fs, was reported by Metzeler et al. [28] Another kinase domain germline variant, D837N, in EGFR was absent in WHISP controls but found in 5/387 ovarian cancer cases with a position matching a reported somatic mutation (D837G) in COSMIC [29] . Germline and somatic interactions in ovarian cancer Since familial cancer predisposition genes are also often somatically mutated in non-familial cases [30] , we examined previously characterized somatic SMGs (and BRCA2 ) that met our expression criteria for putative germline functionally deleterious variants (truncation and predicted deleterious missense) in the germline data of ovarian cancer cases. As expected, a high frequency of germline truncation variants was observed in BRCA1 ( n =32) and BRCA2 ( n =25). We observed one germline truncation variant in NF1 (D290fs) in one case (age of diagnosis: 39 years). We similarly investigated somatically mutated protein tyrosine phosphatases and identified eight germline truncation events in four genes ( PTPN13 , PTPRM , PTPRR and PTPRH ). Notably, four truncation events (two H942fs, one R199fs and one T79fs) were found in PTPRH , a gene not previously linked to ovarian cancer ( Fig. 3 ). Analysis of germline truncations in somatically mutated chromatin modifier genes also identified truncations in SETD4 (Y129fs), SETD6 (M264fs), MLL3 (exon 14-2), SMC5 (Q810fs) and SMC6 (Y954*). This suggests a potential role for histone modifiers in ovarian susceptibility and motivates further study. Predicted functionally deleterious germline missense variants having low frequencies were detected in several somatic SMGs, including BRCA1 (germline missense n =27), BRCA2 ( n =13), NF1 ( n =8), RB1 ( n =3) and TP53 ( n =1; Supplementary Table 3 ). The two patients having a germline V2148D variant in NF1 were diagnosed at ages 36 and 45 years. 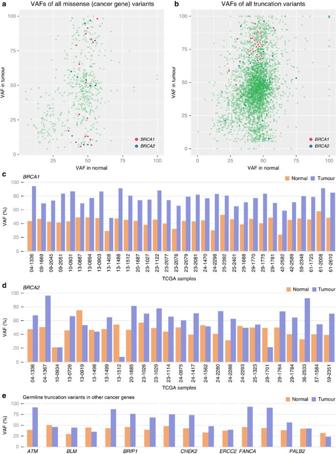Figure 4: LOH analysis in tumour samples. (a) Scatter plot displaying variant allele frequencies for all germline truncation variants in normal and tumour samples. Truncation variants inBRCA1andBRCA2are highlighted in red and blue, respectively. (b) Scatter plot displaying variant allele frequencies for germline missense variants from cancer genes in normal and tumour samples. Germline missense variants inBRCA1andBRCA2are highlighted in red and blue, respectively. (c) VAFs for the 32 samples showing LOH truncation inBRCA1, (d) VAFs for 25 samples showing LOH inBRCA2, (e) VAFs inATM,BLM,BRIP1,CHEK2,ERCC2,FANCAandPALB2.Overall, 100% (32/32) and 76% (19/25) of, respective, germlineBRCA1andBRCA2truncation variants showed increased VAFs in the tumour. All germline truncation variants inBRIP1andCHEK2also showed increased VAFs in corresponding tumours. We further investigated the interplay between germline variants (truncation and missense) and somatic mutations in ovarian cancer, discovering 18 patients with germline truncation variants and somatic mutations in the same gene ( Supplementary Table 4 ). For instance, a patient with a germline frameshift mutation (M723fs) in PALB2 also harboured a somatic nonsense mutation (Q378*) and another patient with a germline nonsense variant (Q153*) in CDK5RAP1 acquired a somatic splice site mutation in that gene (exon 9-2). We also detected eight patients with both germline missense and somatic mutations from the same cancer gene. This list includes two patients with BRCA1 (germline: R1347G and S1512I; somatic: E111* and G813fs), one patient with NF1 (germline: A2644G; somatic: I85fs) and one with TP53 (germline: G334R; somatic: P177R). We investigated LOH in tumour samples for 535 missense variants in cancer genes and 2,214 genes having germline truncation variants (3,635) and found a total of 732 truncation variants (63 in cancer genes) that displayed LOH in the tumour samples (>20% increase of variant allele frequency (VAF) over normal was used for defining LOH, considering the average 77% purity of the ovarian tumour cohort, false discovery rate=22%, Supplementary Fig. 5 and Methods), suggesting their potential roles in ovarian cancer susceptibility ( Fig. 4a,b and Supplementary Data 12 ). Most notably, we observed at least a 20% increased VAF for 30/32 truncation mutations in BRCA1 (all 32 having increased VAFs) and 13/25 in BRCA2 (19 having increased VAFs) in the tumour samples when compared with the paired germline samples ( Fig. 4c,d ). In BRCA1 , 13 LOH events were associated with a loss of one copy in tumour (copy-number segmentation mean ≤1.5), while nine LOH events were associated with a single copy-number loss for BRCA2 . We also identified 14 BRCA1 and 4 BRCA2 copy-number neutral LOH events in tumour samples (1.5<copy-number segmentation mean ≤2.5). A small number of cases carried germline truncation variants with clear evidence of somatic LOH (loss of the wild-type allele) in the tumour samples occurring in genes involved in cell cycle checkpoint, Fanconi/DNA repair pathways (for example, ATM , BRIP1 , CHEK2 , FANCA and MSH3 ), phosphatases (PTPRH and PTPRM) and a putative prostate cancer susceptibility gene, ELAC2 ( Fig. 4e and Supplementary Data 12 ). This evidence suggests that several additional genes may be associated with ovarian cancer susceptibility. Figure 4: LOH analysis in tumour samples. ( a ) Scatter plot displaying variant allele frequencies for all germline truncation variants in normal and tumour samples. Truncation variants in BRCA1 and BRCA2 are highlighted in red and blue, respectively. ( b ) Scatter plot displaying variant allele frequencies for germline missense variants from cancer genes in normal and tumour samples. Germline missense variants in BRCA1 and BRCA2 are highlighted in red and blue, respectively. ( c ) VAFs for the 32 samples showing LOH truncation in BRCA1 , ( d ) VAFs for 25 samples showing LOH in BRCA2 , ( e ) VAFs in ATM , BLM , BRIP1 , CHEK2 , ERCC2 , FANCA and PALB2. Overall, 100% (32/32) and 76% (19/25) of, respective, germline BRCA1 and BRCA2 truncation variants showed increased VAFs in the tumour. All germline truncation variants in BRIP1 and CHEK2 also showed increased VAFs in corresponding tumours. Full size image We examined LOH patterns indicating retained germline missense variants in BRCA1 . Here we identified two known pathogenic missense variants, G1788V and R1699W [31] ( Supplementary Fig. 4 ); R1699W has VAFs of 42 and 79% and G1788V has VAFs of 57 and 98% in the germline and tumour samples, respectively. For one variant of unknown significance, S1521I, evidence indicating loss of the variant allele in the tumour was present in 3/3 cases, suggesting that S1521I is not pathogenic, in agreement with the Breast Cancer Information Core classification [31] . Evidence of LOH was inconsistent for R1347G and R841W with 2/6 and 1/4 cases demonstrating LOH, respectively. Three variants of unknown significance (V772A, P1637L and L668F) identified in single cases showed LOH. The case with the V772A in BRCA1 was diagnosed with ovarian cancer at age of 49 years; however, this case also carried a BRCA1 truncation variant. The case with the V1637L variant in BRCA1 also had a truncation in BRCA2 and V1637L has previously been predicted to be functionally neutral [32] . For L688F that occurred in one ovarian cancer case and was not observed in the WHISP data set, no other truncation mutations were observed. None of the BRCA2 missense variants were classified as clinically important in the Breast Cancer Information Core BRCA2 database [31] , [33] . Evidence of LOH for retaining some germline BRCA2 missense variants (S1172L, T2088I, K2434T and A2951T) was observed ( Fig. 4d ; Supplementary Fig. 4 , and Supplementary Data 13 ). The case harbouring K2434T in BRCA2 was diagnosed at the age of 37 years; however, further work is needed to confirm the functional relevance of such rare germline variants. We expanded our LOH analysis to all rare missense variants across cancer genes (Methods) and identified a total of 114 instances having a greater than 20% increase of VAF in the tumour compared with the germline ( Fig. 4d and Supplementary Data 13 ). We further employed germline–somatic interaction analyses and extensive bioinformatics annotations to identify truncation and missense variants with high likelihood of having functional relevance. Specifically, we examined five aspects of each germline variant (3,635 truncations and 535 missense): pfam annotation, COSMIC/OMIM proximity match, LOH status, somatic SMG status and somatic mutation in the same gene. When limiting our candidates to variants meeting at least two of the five criteria, the numbers of variants with putative functional effects decreased to 302 truncation and 56 missense events, respectively. In addition, we limited our high confidence variants to genes expressed in ovarian cancer (RNA-Seq by expectation-maximization (RSEM)>0.5) and those that had a lower frequency in cases than WHISP controls, thereby obtaining 222 putative variants with functional effects (181 truncations and 41 missense; Table 2 and Supplementary Data 14 ). After removing variants suspected to be non-pathogenic based on previous published findings ( ATM F1463C [34] , BRCA1 L668F and P1637L [32] , PALB2 H1170Y [35] , SMO [36] and TSC2 (refs 37 , 38 )), the missense list includes variants from several genes including the two known pathogenic BRCA1 variants (G1788V and R1699W), four BRIP1 variants, three ATM variants, four NF1 variants and one TP53 variant previously identified in breast cancer [39] ( Table 2 ). Notably, some of the cases with variants identified through this analysis also had truncation variants in known ovarian cancer predisposition genes suggesting an alternative explanation or interacting risk alleles. Our integrated analysis of germline and somatic variants identifies a set of known ovarian cancer susceptibility variants and prioritizes a set of variants without previous association with ovarian cancer susceptibility. Table 2 Thirty-five known and candidate functional missense variants. Full size table Significant pathways in ovarian cancer We performed pathway analysis using PathScan statistical test [40] including both germline truncation variants and somatic mutations and identified the Kyoto Encyclopedia of Genes and Genomes (KEGG) Fanconi anaemia DNA repair pathway as significant ( P =4.2E−08) along with MAPK, cell cycle and TP53 signalling pathways ( Fig. 5 and Supplementary Data 15 ). RB/RAS pathways were previously reported to be involved in ovarian cancer [4] . Germline and somatic mutations in the Fanconi anaemia pathway affected a total of 40 genes in 37% (157/429) cases. Additional rare mutations detected but not shown occurred in APITD1, EME1, ERCC1, HES1, MLH1, PMS2CL, POLK, POLI, RAD51, REV3L, RMI1, RPA1, RPA2, RPA4, TELO2, TOP3A, TOP3B, USP1 and WDR48. 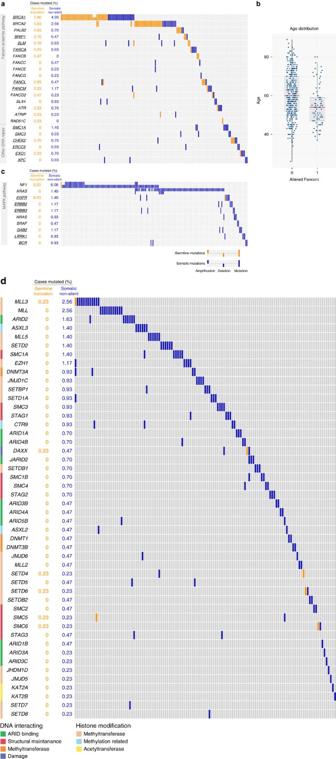Figure 5: Significant pathways and subnetworks in ovarian cancer. (a) Oncoprint of genes with germline truncation variants and somatic mutations found in the Fanconi subnetwork identified as significant by HotNet. Genes in the iRefIndex database58 are underlined. (b) The age distribution for patients with or without germline alterations in Fanconi genes (genes include:a). The horizontal red line indicates the median age of the group and the blue whiskers represent the age of the individual sample. (c) Oncoprint of genes with germline truncation variants and somatic mutations found in the MAPK subnetwork identified as significant by HotNet. Additional genes in the MAPK pathway with somatic mutations and/or germline truncation variants are included. (d) Oncoprint of genes with germline truncation variants and somatic mutations found in a subnetwork includingMLL,MLL3andSETD1Aidentified as significant by HotNet. Additional chromatin modifiers with somatic mutations and/or germline truncation variants are included. Figure 5: Significant pathways and subnetworks in ovarian cancer. ( a ) Oncoprint of genes with germline truncation variants and somatic mutations found in the Fanconi subnetwork identified as significant by HotNet. Genes in the iRefIndex database58 are underlined. ( b ) The age distribution for patients with or without germline alterations in Fanconi genes (genes include: a ). The horizontal red line indicates the median age of the group and the blue whiskers represent the age of the individual sample. ( c ) Oncoprint of genes with germline truncation variants and somatic mutations found in the MAPK subnetwork identified as significant by HotNet. Additional genes in the MAPK pathway with somatic mutations and/or germline truncation variants are included. ( d ) Oncoprint of genes with germline truncation variants and somatic mutations found in a subnetwork including MLL , MLL3 and SETD1A identified as significant by HotNet. Additional chromatin modifiers with somatic mutations and/or germline truncation variants are included. Full size image We used HotNet [41] to identify subnetworks of a genome-scale protein–protein interaction network containing genes with significant numbers of somatic and germline variants. HotNet identified two such subnetworks ( P <0.01): one consisting of DNA repair and Fanconi anaemia genes ( Fig. 5a and Supplementary Table 5 ) that is mutated in 33.1% (142/429) of samples. We combined Fanconi genes from PathScan and HotNet analyses and determined that 40.8% (175/429) of ovarian cancer patients in this study have germline/somatic defects in the Fanconi pathway. As expected, we found that germline alterations in 47 Fanconi genes are significantly enriched in younger patients by a Wilcoxon rank-sum test (427 tumours with data, P -value=1.1878E−05, Fig. 5b ). A second subnetwork containing somatic mutations and germline variants in EGFR , ERRB2 , ERBB3 and other genes is shown in ( Fig. 5c and Supplementary Data 16 ). The frequency of somatic mutations in each of these genes is low (<1.3%), as is the frequency of germline variants (<0.3%). The significance of this subnetwork is thus derived from the combined analyses of somatic mutations, germline variants and biological interactions among these proteins. Using more permissive parameters, HotNet identifies two additional subnetworks (see Methods), including a subnetwork containing MLL , MLL3 and SETD1A ( Fig. 5d and Supplementary Data 16 ). Mutations in these histone methyltransferases have been previously reported in leukemias [42] , breast cancer [24] and renal carcinomas [43] but have not been widely reported in ovarian carcinoma. We report here the first large-scale exome-wide analysis of the combined germline–somatic landscape of ovarian cancer. We used several analytic approaches to sift through millions of germline variants to discover both known and candidate cancer susceptibility genes and loss-of-function truncation and missense variants. As expected, we found enrichment of germline presumed loss-of-function truncation variants in the known ovarian cancer susceptibility genes, BRCA1 , BRCA2 , BRIP1 , CHEK2 and PALB2 . The average diagnosis age for patients with germline BRCA1 / BRCA2 truncation variants was 53.4 years, significantly younger than either patients with somatic BRCA1 / BRCA2 mutations (61.8 years, n =32, P =0.0002, t -test) or the entire cohort (59.4 years, n =427, P= 5.73E−06, t -test). Interestingly, patients harbouring germline BRCA1 / BRCA2 alterations have an average of 1.87 somatic mutations ( n =60) in 127 SMGs from MuSiC analysis of 12 TCGA cancer types [44] (curated from doi:10.1038/nature12634 ), which is markedly lower than patients with somatic BRCA1 / BRCA2 mutations (average of 2.84 somatic mutations, n =32, P =2.1E−05 t -test). Further, likely loss-of-function truncation variants were detected in several other genes/gene family members and syndromes (NF1) that have previously been associated with breast and/or ovarian cancer susceptibility including BLM [15] , FANCD2 (ref. 45 ), NF1 (refs 19 , 46 ), RAD51B [47] , [48] , FANCA [49] , FANCB , FANCL , FANCM , ATRIP and ATR [50] . Notably, loss-of-function variants were dispersed across a set of genes, in particular, previously reported members of the Fanconi pathway [51] and some novel members. The identification of pathogenic missense variants in high-throughput sequencing data is challenging owing to the large number of rare variants of unknown significance and inherent uncertainties associated with in silico -based functional prediction. To identify a set of known and likely pathogenic missense variants, we used several complementary strategies including LOH, COSMIC/OMIM proximity match, PFAM domain and case/control allele frequency analyses. We first applied the LOH analysis to germline truncation variants in BRCA1 and BRCA2 and a small set of other tumour suppressor genes, demonstrating a strong tendency to induce LOH of the wild-type allele in the tumour. For example, clear evidence for LOH of BRCA1 wild-type alleles in the tumour was present in virtually all cases, similar to previous reports [3] , [52] . Further, our analysis identified two pathogenic missense variants (G1788V and R1699W) as well as three with uncertain pathogenicity (L668F, V772A and P1637L) that demonstrated clear evidence of LOH. However, we note that the single cases with V772A and P1637L variants each had a BRCA1 truncation variant suggesting an alternative explanation for these findings. LOH was also observed for several BRCA2 missense variants. Evidence for pathogenicity was also demonstrated for a number of variants in cancer genes including two pathogenic BRCA1 , three ATM and four BRIP1 missense variants that met at least two of the five criteria for classifying candidate pathogenic missense variants. These results emphasize that integration of both somatic and protein domain information can facilitate identification of a set of known and potentially pathogenic missense variants among thousands of rare missense variants that informs functional assessment of variants of unknown significance. Significance analysis of germline truncation and missense variants nominated a set of genes including ASXL1 , MAP3K1 and SETD2 as candidate novel ovarian susceptibility genes. COSMIC somatic mutation matches to ASXL1 germline missense variant (G1397S) coupled with evidence for LOH support a potential role for this variant in ovarian cancer susceptibility. In addition, common variation in MAP3K1 , another member of the MAP3K family, has been associated with breast cancer susceptibility [53] , was recently identified as a target of frequent somatic breast cancer mutations [24] , [25] and was significant based on the burden test. Pathway and network analyses of the integrated collection of germline and somatic variants revealed pathways with significant enrichment of variants including the Fanconi anaemia/DNA repair pathway, MAPK pathway and histone methyltransferases. In most cases, the individual genes in these pathways are altered rarely by either germline or somatic variants, and it is only through the combined analysis of both types of variants across many genes that the alteration of these pathways becomes apparent. This further emphasizes the extensive genetic heterogeneity in serous ovarian carcinoma, as suggested by the relatively small number of genes found to be recurrently mutated by somatic mutations in TCGA study [4] . We are mindful of limitations of TCGA and WHISP data for germline analyses and the analysis of rare variants in general including lack of family history information in TCGA cases that would further inform these results, exclusion of women with a prior malignancy that required systemic therapy from the TCGA case set that might lead to an underestimation of the frequency of germline susceptibility alleles in the population, lack of personal cancer history information in WHISP controls, differences in sequencing platforms used to generate the TCGA and WHISP exome sequence data, and detection of rare germline variants that are extremely rare/private and have no pathogenic significance. With respect to differences in sequencing platforms between the case and control data sets, more variants were called in the WHISP data than the TCGA data, which would reduce our ability to detect significantly higher frequencies of rare deleterious germline variants in TCGA cases compared with WHISP controls. In addition, it is noteworthy that the WHISP controls were older on average than TCGA cases and were assembled for the purpose of examining genetic susceptibility to non-cancer outcomes. Therefore, pathogenic germline variants would most likely be under-represented in this cohort, which would increase our ability to identify pathogenic variants in TCGA ovarian cancer cases. In conclusion, this is the first large scale and comprehensive analysis of both germline and somatic exome variants in ovarian cancer. Our exome-wide analysis strongly supports and extends results from previous studies employing candidate gene approaches for discovery of ovarian cancer genes, and is in line with previous reports by identifying Fanconi anaemia pathway genes as the most frequent targets of germline and somatic mutations. Our integrated analyses of somatic and germline data indicate additional genes and variants of potential importance in ovarian cancer susceptibility for further investigation. In addition, we emphasize that candidate variants and genes nominated by our study will require extensive experimental functional validation as well as replication in additional ovarian cancer datasets. Functionally validated variants will have important implications for the development of screening strategies to evaluate ovarian cancer predisposition. Study population We obtained approval from the database of Genotypes and Phenotypes (dbGaP) to access the exome sequence and clinical data from TCGA ovarian cancer cases for this study (document number 3281 Discover germline cancer predisposition variants). We selected a total of 460 ovarian cancer cases (316 cases previously reported [4] and 144 new ovarian cases) with their germline and tumour DNA sequenced by exome capture followed by next-generation sequencing on Illumina or SOLiD platforms. Of the 460 cases, 429 met our inclusion criteria of 50% coverage of targeted exome having at least 20 × coverage in both germline and tumour samples. Seventy-four percent of targets reached 20 × coverage for 80% of breadth. Population estimates of allele frequencies were obtained from a control group of 3,505 European individuals from the NHLBI exome data set ( https://esp.gs.washington.edu/drupal/ ), and from 379 European, 246 African, 286 ASN and 181 AMR descent individuals from the 1,000 genomes project [54] . The global MAFs were obtained from the single nucleotide polymorphism (SNP) database release 137, based on the 1,000 genomes phase 1 genotypes for 1,094 individuals, released on May 2011. Ancestry classification using PLINK TCGA ovarian cancer cases were classified with respect to ancestry using their SNP array data [4] and the multi-dimensional scaling analysis program in PLINK (http://pngu.mgh.harvard.edu/~purcell/plink/ , version 1.07). Five clusters were used for multi-dimensional scaling analysis. Twenty-three TCGA cases had unknown ethnicity information; we were able to assign ethnicity for 19 of these as Caucasian ( n =17) and African American ( n =2) using principal components analysis ( Supplementary Fig. 1 ). Control cohort WHISP data for 614 samples were downloaded from dbGaP (dbGaP Study Accession: phs000281.v4.p2), verified for file integrity, and then imported as BAM files into our data warehouse. The WHISP data were collected as part of the NHBLI Exome Sequencing Project that has the objective of detecting genetic variants related to heart, lung and blood diseases as described at http://www.ncbi.nlm.nih.gov/projects/gap/cgi-bin/study.cgi?study_id=phs000281.v4.p2 . Women included in WHISP were a subset of women who were part of the Women’s Health Initiative [55] . To minimize batch differences between the ovarian data set and these controls, we processed imported samples through the same pipeline, including alignment to the GRCh37-lite reference sequence with BWA [56] v0.5.9 with parameters –t 4 –q 5 and marking of duplicates by Picard v1.46. Single nucleotide variants (SNVs) and indels were called using VarScan v2.2.9 (with parameters --min-coverage 3 --min-var-freq 0.20 -- P -value 0.10 --strand-filter 1 --map-quality 10) with the false-positive filter [57] and GATK [58] v5336 (with parameters -T IndelGenotyperV2 --window_size 300). Variant calls were restricted to the ~34 Mbp CDS target region [4] . To remove outliers in data quality, we required that WHISP samples have read mapping rates <80%, duplication rates <40% and at least 10,000 SNVs called in the target region. The 557 WHISP samples that met these criteria had, on average, mapping rates of ~95%, duplication rates of ~9% and ~18,000 SNVs called in the target region. Eighty-one percent of targets reached 20 × coverage for 80% of breadth. These were used as controls in the downstream analysis. Germline variant calling and filtering Sequence data from paired tumour and germline samples were aligned independently to NCBI Build 36 of the human reference using BWA 0.5.9 and de-duplicated using Picard 1.29. Germline SNPs and indels were identified in paired BAMs using VarScan2 with the following parameters: min-coverage=30, min-var-freq=0.08, normal-purity=1, P -value=0.10, somatic- P -value=0.001 and validation=1. Additional germline SNPs were identified using Samtools (version 0.1.7a (revision number 599) and additional germline indels were identified using GATK (version 1.0 (revision 5336). All predicted variants were filtered to remove false positives related to potential homopolymer artifacts (variants found in homopolymers having sequence length ≥5 were removed), strand-specific sequence artifacts, ambiguously mapped data (average mapping quality difference between the reference supporting reads and variant supporting reads ≥30) and low quality data at the beginning and end of reads (variants supported exclusively by bases observed in first or last 10% of the reads). Variants having an allele frequency <8% were removed. Initial variant transcript annotation was based on a combined database, including NCBI Refseq (May 2009) and Ensembl (version 54). All variants were additionally annotated using (version 2.2) of Ensembl Variant Effect Predictor [59] . Variants that occurred outside tier 1 (coding exons, canonical splice sites and RNA genes) and variants that did not change the amino-acid sequence were not included in the downstream analysis. Putative variants with translational effect were filtered in the multistep process shown in Supplementary Fig. 2 and described below. Variants were filtered if they either could not be mapped uniquely from NCBI build 36 to GRCh37, were protein altering in a rare transcript that was exclusive to either the NCBI or Ensembl database, or if they were non-synonymous only in transcripts that lacked a valid open reading frame due to internal frame shifts, missing start codons and/or missing stop codons. In addition, all variants were discarded from genes suspected to have pseudogenes or other prologues missing from the human reference sequence, such as PDE4DIP , CDC27 , MUC4 , DUX4 and XPC . We additionally filtered variants that occurred exclusively in non-coding RNA genes, those that affected only predicted, hypothetical or olfactory genes, those that had a frequency>1% in the Caucasian population in the NHLBI GO exomes sequence data, those exclusively within a transcript annotated as a pseudogene or processed pseudogene based on Ensembl release (64) annotation downloaded via Biomart and finally those that were reported as a validated somatic mutation in the same sample. Sequence data supporting all remaining germline truncational variants were visually examined with the Integrative Genomics Viewer [60] and any data that appeared to be supported by potential sequencing, amplification or alignment artifacts were discarded. Additional validated germline variants reported in BRCA1 , BRCA2 were recovered, followed by removal (filtering) of any remaining non-synonymous germline variants that were recurrent at the same position in more than 2% of the cohort (more than eight samples at the same position). Finally, for the analysis of SMGs, genes not typically expressed in ovarian adenocarcinoma tumour samples were filtered if they had an average RPKM ≤0.5. For the RNA-seq-based gene expression analysis, we used the Pancan12 per-sample log2-RSEM matrix from doi:10.7303/syn1734155.1 . A gene qualified as expressed if it had at least three reads in at least 70% of samples. For every gene, the average per-sample RSEM value was calculated across samples from the same tumour type. The genes that had an average RSEM<0.5% were considered to be low-expressed genes. Of the 20,239 genes that had an expression value in ovarian cancer, 4,957 were low-expressed genes. Cancer gene list The cancer gene list ( Supplementary Data 17 ) comprised of a total of 672 unique genes of interest that included 436 genes from the Sanger Cancer Gene [9] list ( http://www.sanger.ac.uk/genetics/CGP/Census/ as downloaded on 1 December 2010), 41 uterine and endometrial cancer genes that we previously identified as having recurrent somatic mutations [12] and 50 genes that have been identified in genome-wide association studies as containing common cancer susceptibility variants to ovarian or breast cancer (HugeNet, http://www.cdc.gov/genomics/about/index.htm ). Of note, the 436 genes on the Sanger cancer gene list contained gene clusters (IGH@, IGK@ and IGL@). Individual genes from these clusters were extracted. Any genes on the list that represented common fusion products of translocation or any gene that could not be identified based on Ensembl release 58 and the corresponding release of NCBI Refseq from the same time point were excluded. This process resulted in a total of 616 putative cancer-related genes. Validation of truncation variants in cancer genes We designed validation PCR primers pairs using Primer3 and tailed the sequences with universal forward and reverse primer sites. Primer pairs for PCR were selected to favour products with an optimal size of 200–300 bp. ( Supplementary Data 19 and 20 ) Larger or smaller products were allowed to avoid problematic sequences. Alternate sources of whole genome amplified (WGA) or original source genomic DNA samples from tumour and normal pairs were amplified with PCR using a single-primer pair and each individual PCR product was sequenced with BigDye Terminators using universal primers. Products were purified and then loaded on an ABI 3730. Resulting reads were base called using Phred, and aligned to genomic sequence representative of the PCR products using Crossmatch. PolyScan [61] and PolyPhred [62] were used to identify SNPs and Indels. Predicted putative rare germline variants were visually reviewed using Consed to determine the exact position and sequence of indel events and eliminate false positives due to data quality, LOH in the tumour sample, artifacts resulting from sequence context, paralogue amplification, or WGA or Illumina library generation or sequencing artifacts. Missense germline variant analysis Missense germline variants were filtered using the same methods ( Supplementary Fig. 3 ) previously described for germline truncations. To minimize the number of variants tied with ancestral origins, only missense germline variants from individuals classified as Caucasian by Plink were used for downstream significance testing. Missense germline variants were further filtered to retain only those identified as deleterious by the Ensembl implementation of Condel, a software program that employs a weighted approach to calculate the functional impact of missense variants from scores calculated by SIFT [63] and PolyPhen-2 (ref. 64 ). We then removed missense germline variants that occurred at >1% frequency in the ovarian cancer cases and followed that by removing germline predicted missense variants that were better classified as somatic variants. Variants with population MAFs ≥1% in NHLBI ESP GO exomes or 1,000 genomes were also filtered. Remaining sites were annotated using the Ensembl variant effect predictor instance of Condel and remaining predicted deleterious variants were retained for burden analysis. Sites were further filtered to only retain expressed variants in cancer genes (as described above). In addition, we have performed internal unbiased validation of all rare variants identified in 11 cases using available whole-genome sequencing data that were independently generated. It is noteworthy that whole-genome sequencing data for two cases were generated using the SOLiD platform, furnishing orthogonal validation of the variants discovered using Illumina sequencing data. ( Supplementary Data 18 ). We applied a modified version of the CAST [11] to the final list of germline missense variants in the ovarian cancer data set to determine the statistical significance of deleterious variants in genes that were over-represented in ovarian cases versus control exomes from the WHISP. A one-tailed CAST test was used to identify only the genes with higher burden frequency in cases than in controls. Germline copy-number alterations analysis Segmented copy-number deletion events were extracted from GISTIC (10.1073/pnas.0710052104) analysis of Affymetrix 6.0 SNP array data for a total of 426 exome sequenced tumour-normal sample pairs with available array genotype data. Matched tumour and normal samples were processed in parallel to identify putative germline copy-number variations (CNV) with overlapping deletion segments defined by eight consecutive probes in both tumour and normal. Potentially truncating CNV deletion events in the 672 cancer-related genes list were extracted from the total list. Graphical plots were visually examined to identify and filter suspected artifacts and somatic copy-number events. All CNV deletion events were annotated to identify those overlapping coding exons and those that were intronic, intergenic, or affected untranslated region exons were removed. Matched tumour-normal exome capture BAMs were examined to identify any heterozygous SNPs refuting germline copy-number deletions or, alternatively, to identify coverage anomalies supporting the presence of germline deletion events. Finally, individual probe intensities were plotted and reviewed to remove additional artifacts. LOH analysis LOH analysis was performed by calculating the VAF of both SNV and short indels using our internally developed tool bam-readcount ( https://github.com/genome/bam-readcount ) for SNVs and Samtools mpileup [6] /VarScan [7] for indels. Significance testing was done on the basis of generating an approximate empirical distribution of the actual population null distribution using a resampling method (bootstrapping with replacement). We corrected each case for tumour purity using where VAF tumour,C and VAF tumour,U are the corrected and uncorrected tumour variant allele fractions, respectively, P tumour is tumour purity and VAF normal is variant allele fraction in the normal. This equation is an algebraic consequence of assuming that foreign variant and reference reads in the tumour are proportional to their corresponding numbers in the normal sample. The distribution converged within 10 8 trials ( Supplementary Fig. S4 ) and this, in turn, agreed well with another distribution model obtained by full enumeration of all possible VAF differences within the data set. A threshold of 20, that is, P tumour × (VAF tumour –VAF normal ) ≥20%, was taken as significant and this threshold incurs a false-positive error rate of roughly α =22%. The actual error rate may be slightly less because VAF differences above 50 are, strictly speaking, spurious and probably due to contamination in the normal. Pathway analysis using HotNet We applied HotNet [65] to identify subnetworks in a genome-scale protein–protein interaction network, each containing genes with significant numbers of somatic and germline aberrations. HotNet identifies a list of subnetworks, each containing at least s genes, and employs a two-stage statistical test to assess the significance of the list of subnetworks. We used HotNet version 1.1 and an interaction network from iRefIndex 9 (ref. 66 ) containing 212,746 interactions among 14,384 proteins, using parameter t =0.05 to derive the influence graph. With parameter δ =0.02, we find two subnetworks ( Supplementary Table 5 ), each containing at least six genes ( P =0.0005). With parameter δ =0.02, we find four subnetworks ( Supplementary Data 16 ), each containing at least four genes ( P =0.1555). How to cite this article: Kanchi, K. L. et al. Integrated analysis of germline and somatic variants in ovarian cancer. Nat. Commun. 5:3156 doi: 10.1038/ncomms4156 (2014).